Textured fluorapatite bonded to calcium sulphate strengthen stomatopod raptorial appendages Stomatopods are shallow-water crustaceans that employ powerful dactyl appendages to hunt their prey. Deployed at high velocities, these hammer-like clubs or spear-like devices are able to inflict substantial impact forces. Here we demonstrate that dactyl impact surfaces consist of a finely-tuned mineral gradient, with fluorapatite substituting amorphous apatite towards the outer surface. Raman spectroscopy measurements show that calcium sulphate, previously not reported in mechanically active biotools, is co-localized with fluorapatite. Ab initio computations suggest that fluorapatite/calcium sulphate interfaces provide binding stability and promote the disordered-to-ordered transition of fluorapatite. Nanomechanical measurements show that fluorapatite crystalline orientation correlates with an anisotropic stiffness response and indicate significant differences in the fracture tolerance between the two types of appendages. Our findings shed new light on the crystallochemical and microstructural strategies allowing these intriguing biotools to optimize impact forces, providing physicochemical information that could be translated towards the synthesis of impact-resistant functional materials and coatings. Stomatopods, or ‘mantis shrimps’, are crustaceans that have evolved a pair of powerful raptorial appendage used during their aggressive hunting strategies. These intriguing structures can take two forms depending on the species: a ‘smasher’ ( Fig. 1a ) that is used as an impact hammer to shatter hard shells and incapacitate their prey, or a ‘spear’ that serves as a grasping and holding device for passing prey ( Fig. 1e ). In addition to being used to grasp and impale their prey, at close proximities, the spear-like modification can be used in a hammer-like fashion and possesses a distinctive flattened impact surface. Both limbs are deployed at a remarkably high velocity of up to 23 m s −1 , which represents one of the fastest appendage movements in the animal kingdom [1] . Recent investigations by Weaver et al. [2] have revealed the complex interplay between microstructure, mechanical properties and impact mechanics of the dactyl club from Odontodactylus scyllaru s. These findings have showed that the club is divided into three distinct regions: (i) the impact surface made of highly crystalline apatite and that is near or in direct contact with the external environment, (ii) the periodic region made of a rotated plywood of chitin/amorphous calcium carbonate (ACC) whose main role is to protect the tool against internal damage, and (iii) the striated region made of mineralized chitin fibrils running in a nested fashion around the club, which presumably prevents expansion during impact. 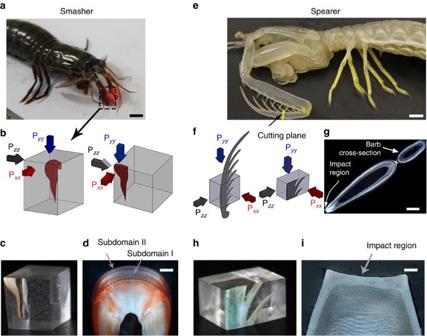Figure 1: Stomatopod dactyl club and spear macro- and microstructures. (a) (Scale bar, 1 cm) Anterior view of a ‘Smasher’-type stomatopod with extended dactyl clubs. (b) Schematic of sample preparation before and after polishing. (c) Overview photograph of the mounted sample after polishing. (d) (Scale bar, 500 μm) Optical micrograph of a yy cross-section showing the two subdomains of the impact region. (e) (Scale bar, 1 cm) Anterior view of a ‘Spearer’-type stomatopod with a single visibly extended appendage. (f) Schematic of sample preparation for indentation and spectroscopic measurements. (g) (Scale bar, 500 μm) Optical micrograph of a yy cross-section illustrating the location of the impact region. (h) Overview photograph of the mounted sample after polishing. (i) (Scale bar, 50 μm) Higher magnification micrograph of the impact region of (g).Piirefers to nanoindentation experiments performed perpendicular to the ii plane. Figure 1: Stomatopod dactyl club and spear macro- and microstructures. ( a ) (Scale bar, 1 cm) Anterior view of a ‘Smasher’-type stomatopod with extended dactyl clubs. ( b ) Schematic of sample preparation before and after polishing. ( c ) Overview photograph of the mounted sample after polishing. ( d ) (Scale bar, 500 μm) Optical micrograph of a yy cross-section showing the two subdomains of the impact region. ( e ) (Scale bar, 1 cm) Anterior view of a ‘Spearer’-type stomatopod with a single visibly extended appendage. ( f ) Schematic of sample preparation for indentation and spectroscopic measurements. ( g ) (Scale bar, 500 μm) Optical micrograph of a yy cross-section illustrating the location of the impact region. ( h ) Overview photograph of the mounted sample after polishing. ( i ) (Scale bar, 50 μm) Higher magnification micrograph of the impact region of ( g ). P ii refers to nanoindentation experiments performed perpendicular to the ii plane. Full size image The impact surface is critical particularly for the hunting success of stomatopods, since its role is to inflict an impact force as high as possible during a single blow. To assist in this function, species have developed both chemical and microstructural strategies in their evolutionary toolkit. Ultra-high mineralization [3] , [4] is an obvious choice to optimize the hardness and stiffness near free surfaces, and most species indeed fine-tune the biomineralization process such that the mineral phase at the free surface exhibits a combination of mechanical properties that is optimized for impact or abrasion tolerance [5] , [6] . Illustrative examples of this strategy include, among others, protective scales of fish [7] , the chiton radular teeth [8] or the external protective armour of deep-sea gastropods [9] . Microstructural adjustments are also commonly employed by species as a way to provide an extra level of control over the properties of their extracellular tissues and tools, with specific examples including porosity gradients in bones [10] or the preferred crystalline orientation in both vertebrate and invertebrate teeth [11] . Stomatopods employ both strategies in their dactyl clubs. Moving from the bulk of the club to its surface, it was found that amorphous calcium carbonate is gradually replaced by amorphous calcium phosphate, which is itself progressively substituted by hyper-mineralized calcium phosphate, with nanoindentation data distinctly showing that this chemical gradation correlates with elastic modulus and hardness ones. Synchrotron X-ray mapping indicated that the apatite crystallites are preferentially oriented with their long axis perpendicular to the surface or equivalently parallel to the loading direction during impact. Here we investigated the impact surface in more detail using confocal Raman microscopy, polarized light microscopy, energy dispersive spectroscopy (EDS) mapping, electron probe micro analyser (EPMA), multidirectional depth-sensing nanoindentation and indentation fracture studies with the goal to elucidate the relationships between mineral phase distribution and texture with the microscale mechanical properties. By the use of these combined techniques, we were able to identify two new impact-region-specific crystalline phases that were not previously detected in stomatopod dactyl segments, namely fluorapatite (FAP) and calcium sulphate (CAS), with the former progressively substituting amorphous calcium phosphate (ACP) closer to the impact surface. Ab initio computations of the FAP/CAS interface suggest that the two minerals are stabilized by a network of hydrogen bonding, with a greater binding energy than computed for hydroxyapatite (HAP)/CAS interfaces. Nanomechanical data also reveal clear evidences of elastic modulus and hardness anisotropy in the impact region for both types of species (the smashers and the spearers), with the highest values measured normal to the impact surface. Our results imply that fluorine substitution for hydroxyls in the apatite crystal lattice is an important parameter in endowing stomatopod-hunting appendages with optimal mechanical and surface chemistry properties, that CAS provides additional mechanical and chemical stability and that the preferred crystallite orientation correlates with stiffness and hardness anisotropy. Finally, indentation fracture studies indicate a higher damage tolerance for the smasher type of stomatopods, which is attributed to the residual organic chitin phase in the impact region that is absent in the spearer species. Microstructural features and preferred fibre orientation Optical micrographs of a spearer sample (yy cross-sectional plane, Fig. 2a,b ) show a clear distinction between the bulk material and the impact region, which can also be discerned on low-magnification field emission scanning electron microscopy (FESEM) images ( Fig. 3a,b ). The bulk material is made of successive layers about 10–50 μm thick with an orientation that follows the outer contour of the cross-section. The impact region is about 50 μm thick at the centre of the region but decreases on the sides. In the smasher species, the impact region is divided into two subdomains ( Fig. 1d ). Subdomain I, which is adjacent to the periodic region of the bulk, is about 500–700 μm thick, and exhibits elastic modulus ( E ) and hardness ( H ) values of 45 and 1.8 GPa [2] , respectively. Subdomain II is thinner (about 50 μm thick) and expands towards the impact surface, with E and H values sharply increasing from subdomain I. 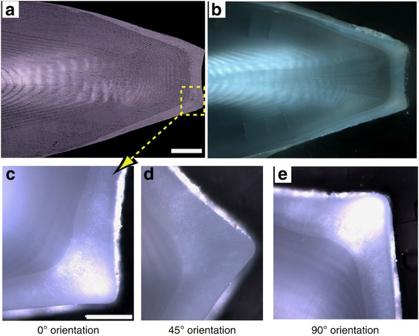Figure 2: Optical micrographs of spearing appendage (yycross-section). (a) (Scale bar, 100 μm) Bright field image. (b) Polarized light image. (c–e) (Scale bar, 50 μm) Polarized light micrographs at various sample rotations. Note the apex region appearing bright at 0° and 90° orientations, and in dark at a 45° orientation. Figure 2: Optical micrographs of spearing appendage ( yy cross-section). ( a ) (Scale bar, 100 μm) Bright field image. ( b ) Polarized light image. ( c – e ) (Scale bar, 50 μm) Polarized light micrographs at various sample rotations. Note the apex region appearing bright at 0° and 90° orientations, and in dark at a 45° orientation. 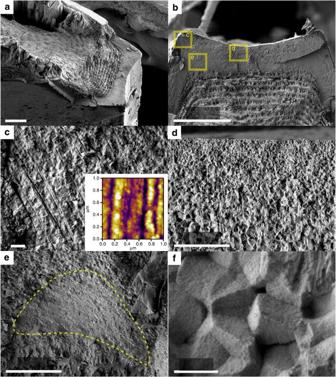Figure 3: FESEM micrographs of the impact region fracture surface from a spearing appendage. (a) (Scale bar, 100 μm) Low-magnification side view and (b) (Scale bar, 100 μm) top view of the impact region. (c) (Scale bar, 1 μm) High-magnification view of the apex region, which is subjected to the highest impact forces, showing the elongated bundle of crystallites between adjacent channel-like structures. Inset: atomic force microscope zoom-in illustrating the lamellar microstructure with lamellae 50–200 nm thick. (d,f) (Scale bar (d), 10 μm, Scale bar (f) 1 μm) High-magnification views of the centre of the impact region showing the presence of equiaxed crystallites as opposed to elongated fibres observed in (c). Note that the crystallite size decreases towards the outer surface. (e) (Scale bar, 10 μm) Subregion of the impact region with a contour line highlighting regions where no crystallites are observed. All features described were consistently observed on various samples. Full size image Figure 3: FESEM micrographs of the impact region fracture surface from a spearing appendage. ( a ) (Scale bar, 100 μm) Low-magnification side view and ( b ) (Scale bar, 100 μm) top view of the impact region. ( c ) (Scale bar, 1 μm) High-magnification view of the apex region, which is subjected to the highest impact forces, showing the elongated bundle of crystallites between adjacent channel-like structures. Inset: atomic force microscope zoom-in illustrating the lamellar microstructure with lamellae 50–200 nm thick. ( d , f ) (Scale bar ( d ), 10 μm, Scale bar ( f ) 1 μm) High-magnification views of the centre of the impact region showing the presence of equiaxed crystallites as opposed to elongated fibres observed in ( c ). Note that the crystallite size decreases towards the outer surface. ( e ) (Scale bar, 10 μm) Subregion of the impact region with a contour line highlighting regions where no crystallites are observed. All features described were consistently observed on various samples. Full size image Optical micrographs, shown in Fig. 2a,b in bright and dark field, respectively, further reveal that the spear impact region exhibits two symmetrical extruded edges on each side of the cross-section. Because of this extruded geometry, these edges must be subjected to the highest contact forces during impact or grasping. Polarized light microscopy imaging reveals that the edges are birefringent, as revealed by the bright and dark contrast at sample/analyser orientations of 0° and 90° and 45°, respectively ( Fig. 2c–e ), which is suggestive of a fibrous or lamellar micro- and nanostructure in biological materials [12] . FESEM studies of a spear fracture surface confirm this hypothesis. At high magnifications ( Fig. 3c ), a fibrous/lamellar microstructure is observed, with a preferred lamellar orientation perpendicular to the outer surface. Further evidence of the fibrous/lamellar structure of the edges was obtained by imaging a polished sample by AFM (inset), which confirms the fibrous structure of the edge with fibrous/lamellar features measuring 50–200 nm thick. This is stark contrast with the centre of the impact region ( Fig. 3d,f ), which exhibits equiaxed crystallites with no preferred orientation. A noteworthy feature of these crystallites is that their size clearly decreases towards the outer surface by nearly 10-fold, with an average size of 100–200 nm near the bulk down to 10–30 nm at the surface. Investigations by synchrotron X-ray diffraction on the smasher clubs had previously indicated that the apatite crystallites are preferentially oriented perpendicular to the surface near the impact region. Chemical mapping and gradients EDS elemental mapping (Ca, P, C, Mg, S, F) of a spear sample cross-section ( Fig. 4 ) shows that Ca and Mg ( Fig. 4b,f ) are all present in significant concentrations, whereas C ( Fig. 4d ) is detected in relatively small amounts. These results are analogous to the previous data reported for O. scyllarus club samples, where the bulk region was found to be mainly comprised of ACC with Mg playing a role of stabilizing the amorphous over the crystalline carbonate [13] . Mapping in the impact region over much longer time durations, however, provides further important findings. In addition to the high phosphorous concentration ( Fig. 4c ), sulphur and fluorine ( Fig. 4g,h ) signals are also detected, with the S mapping showing enriched regions along the contour of the impact region. S and F are similarly distributed in the club samples ( Supplementary Fig. 1 ). Since EDS is only semi-quantitative for light elements, we used EPMA to obtain quantitative elemental analysis ( Supplementary Table 1 ). The C content decreases from ca . 17 at. pct in the bulk to 7 at. pct in the impact regions. In contrast, the S content is four- to fivefold higher in the impact regions, suggesting that sulphur is not associated with residual organic material. This finding is further confirmed by the Raman spectroscopy data. 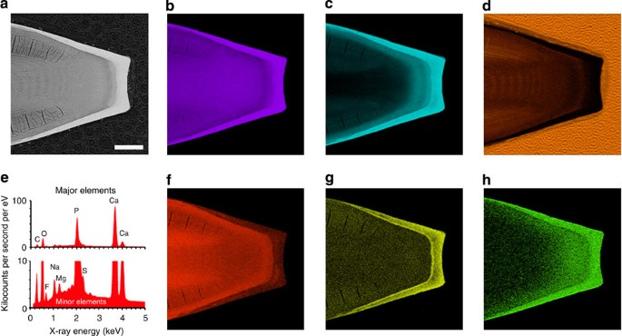Figure 4: EDS elemental maps of a sectioned and polished spearing dactyl segment. (a) (Scale bar, 100 μm) Backscattered electron micrograph revealing the local differences in electron density (yycross-section). (b) Calcium. (c) Phosphorous. (d) Carbon. (e) Point spectrum acquired in the impact region. (f) Magnesium. (g) Sulphur. (h) Fluorine. All maps were background subtracted. Figure 4: EDS elemental maps of a sectioned and polished spearing dactyl segment. ( a ) (Scale bar, 100 μm) Backscattered electron micrograph revealing the local differences in electron density ( yy cross-section). ( b ) Calcium. ( c ) Phosphorous. ( d ) Carbon. ( e ) Point spectrum acquired in the impact region. ( f ) Magnesium. ( g ) Sulphur. ( h ) Fluorine. All maps were background subtracted. Full size image Raman spectroscopy profiles (range 800–1,200 cm −1 ) from the bulk to the surface region ( Fig. 5a , spear sample) indicate the following salient features. In the bulk, ACC is the main band detected (trace i), but the ACC intensity decreases towards the impact region (trace ii). Amorphous calcium phosphate (ACP) exhibits an opposite trend, namely, a low-intensity peak appearing deep in the bulk which becomes the dominant peak close to the bulk-impact region interface. Approaching the free impact surface, the carbonate band diminishes, whereas the phosphate peak sharpens significantly (trace iii)—indicative of higher crystallinity—and shifts towards 965 cm −1 , which is associated with FAP [14] . A sulphate band (1,007 cm −1 ) is also observed in the impact surface region. Raman spectra profiles of the club sample ( Fig. 5b ) show identical trends. EDS and EPMA elemental data as well as Raman spectroscopy analysis thus indicate that the outer layer is composed of FAP instead of HAP, which was previously not distinguishable by X-ray diffraction analysis of the (002) reflection, and that a sulphate phase is also present in the appendages. Known sulphated biominerals include the hydrated CAS gypsum (CaSO 4 ·2 H 2 O), barite (barium sulphate, BaSO 4 ) and celestite (strontium sulphate, SrSO 4 ) [15] . In EDS area elemental analyses, Ba is not found anywhere in the clubs, whereas trace amount of Sr is detected, but with little variation for both the bulk and the impact regions ( Supplementary Fig. 2 ). With EPMA, neither Ba nor Sr is found ( Supplementary Table 1 ), whereas the S concentration is four- to fivefold higher in the impact regions. These data suggest that trace amount of Sr is substituted for Ca in the apatite lattice, but not associated with sulphate. A further confirmation of the source of the sulphate phase is obtained by inspecting the Raman shifts associated with the SO 4 2− ν 1 symmetric mode. For gypsum, barite and celestite, these bands are centred at 1,008, 989 and 1,000 cm −1 , respectively [16] , [17] , [18] . In our measurements, the Raman shift is located at 1,007–1,008 cm −1 . Taken together, these spectroscopic data lead us to conclude that the sulphated compound in the clubs is CAS. The ν 1 mode also provides additional information about the level of hydration of the CaSO 4 phase; partially dehydrated bassanite (CaSO 4 ·0.5 H 2 O) and anhydrite (CaSO 4 ) are centred at 1,015 and 1,017 cm −1 , respectively [16] , thus implying that the CAS phase is the hydrated gypsum. 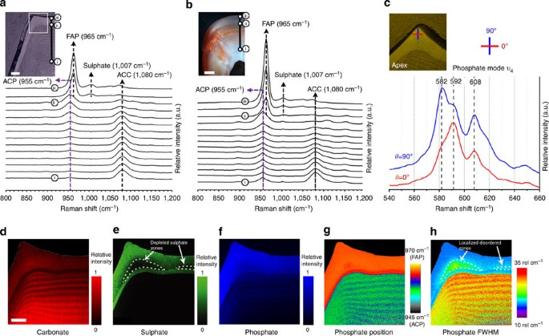Figure 5: Raman spectra profiles from bulk to impact surface. Raman profiles with a range 800–1,200 cm−1. (a) (Scale bar, 50 μm) Spearing and (b) (Scale bar, 500 μm) smashing dactyl segments. Broad band centred at 1,080 cm−1: amorphous calcium carbonate (ACC). Band centred at 955 cm−1: amorphous calcium phosphate (ACP). Sharp band shifted towards 965 cm−1: crystalline fluorapatite (FAP). Comparison with fluorine EDS maps (Fig. 4h) suggests that ACP is also predominantly fluorinated. Band at 1,007 cm−1(only found in the impact region): calcium sulphate (CAS, gypsum). (c) Polarized Raman spectra (range 540–660 cm−1) acquired in the apex region with polarization angles of 0° and 90° relative to the free surface. (d–h) Raman mapping of the spear impact surface with a box in (a) highlighting the region where Raman mapping was carried out. (d) (Scale bar, 30 μm) Carbonate intensity. (e) Sulphate intensity. (f) Phosphate intensity (full phosphate band, with centre of Gaussian fit adjusted for integration). (g) Centre of phosphate peak showing a clear shift at the interface from ACP to FAP. (h) Full width at half maximum (FWHM) of the phosphate band, with lower values indicating crystalline FAP and higher values indicating disordered ACP phase. Note that high crystallinity of FAP is co-localized with the sulphate intensity in the impact region and vice versa. Figure 5: Raman spectra profiles from bulk to impact surface. Raman profiles with a range 800–1,200 cm −1 . ( a ) (Scale bar, 50 μm) Spearing and ( b ) (Scale bar, 500 μm) smashing dactyl segments. Broad band centred at 1,080 cm −1 : amorphous calcium carbonate (ACC). Band centred at 955 cm −1 : amorphous calcium phosphate (ACP). Sharp band shifted towards 965 cm −1 : crystalline fluorapatite (FAP). Comparison with fluorine EDS maps ( Fig. 4h ) suggests that ACP is also predominantly fluorinated. Band at 1,007 cm −1 (only found in the impact region): calcium sulphate (CAS, gypsum). ( c ) Polarized Raman spectra (range 540–660 cm −1 ) acquired in the apex region with polarization angles of 0° and 90° relative to the free surface. ( d – h ) Raman mapping of the spear impact surface with a box in ( a ) highlighting the region where Raman mapping was carried out. ( d ) (Scale bar, 30 μm) Carbonate intensity. ( e ) Sulphate intensity. ( f ) Phosphate intensity (full phosphate band, with centre of Gaussian fit adjusted for integration). ( g ) Centre of phosphate peak showing a clear shift at the interface from ACP to FAP. ( h ) Full width at half maximum (FWHM) of the phosphate band, with lower values indicating crystalline FAP and higher values indicating disordered ACP phase. Note that high crystallinity of FAP is co-localized with the sulphate intensity in the impact region and vice versa. Full size image Polarized Raman measurements in the impact region at 0° and 90° polarization angles relative to the free surface were also conducted. Salient features of these spectra in the range 540–660 cm −1 ( Fig. 5c ) are the presence of two maxima at 582 and 592 cm −1 attributed to the ν 4 phosphate vibration mode [19] and displaying opposite intensity trends. The 582 cm −1 peak is the most intense at 90°, whereas at 0° the maximum intensity shifts towards the 592 cm −1 peak. Finally, Raman spectra of the impact region were also acquired on three mutually perpendicular surfaces prepared according to Fig. 1f (which are identical to the surfaces probed by nanoindentation described in the next section). The relative intensity of the main FAP peak centred at 965 cm −1 is slightly lower when probed in the zz direction as compared with the yy direction, whereas the relative intensity of the 1,073 cm −1 peak exhibits an opposite trend with a higher intensity in the zz direction ( Supplementary Fig. 3 ). To better visualize the distribution of the various phases, we performed confocal Raman imaging ( Fig. 5d–h and Supplementary Fig. 4 ). Not surprisingly, the carbonate ( Fig. 5d ) is the dominant mineral phase in the bulk, mostly in an amorphous form. Interestingly, the carbonate map also indicates a periodicity that follows the layered structure observed by optical microscopy and SEM. The overall phosphate distribution ( Fig. 5f ) unambiguously shows a higher relative intensity of phosphate in the impact region. The spatial discrimination between ACP and FAP was assessed by mapping the spectral position of the centre of the phosphate band ( Fig. 5g ). The resulting map clearly shows that the phosphate band is centred at 955 cm −1 throughout the bulk, whereas the entire impact region is centred at 965 cm −1 , corresponding to FAP. The interface between the two regions appears to be steep as visually illustrated by the sudden colour change from green to red. The full width at half maximum (FWHM) of the phosphate band, which can be related to phase crystallinity ( Fig. 5h ), further indicates that the peak is sharper in the impact region, indicating higher crystallinity of the FAP phase. Sulphate band integration was also performed ( Fig. 5e ) and shows that sulphate is only present in the impact region and is co-localized with the FAP. Further, subtle details emerge by comparing the sulphate with the carbonate and phosphate distributions: a higher relative intensity of the sulphate peak is observed in a strip region ~10 μm thick directly adjacent to the bulk, and this correlates with an almost zero intensity of the carbonate band. In addition, depleted zones (contour highlighted in Fig. 5e ) of the sulphate distribution within the impact region correlate with a local decrease of crystallinity of the phosphate phase (highlighted green/yellow zone of FWHM map in Fig. 5h ). These regions are also characterized by a higher content of carbonate ( Fig. 5d ) and Mg ( Fig. 4f ). Under high-resolution FESEM ( Fig. 3e ), this zone also features a clear microstructural distinction in comparison to the regions that are characterized by a sharp FWHM, with no crystallites observed where the CAS intensity is low. Taken together, the data suggest that enriched sulphate concentration directly correlates with higher crystallinity of the FAP and that inversely, depleted sulphate patches together with higher carbonate and Mg content, decrease FAP crystallinity. In addition, electron diffraction analyses by transmission electron microscopy (TEM) also confirmed the presence of both crystalline and amorphous domains in the impact regions ( Supplementary Note 1 ), with crystalline reflections that could be assigned to both FAP and CAS. TEM investigations are useful to distinguish crystalline from amorphous regions of biominerals in the submicrometer length scale [20] , [21] ; however, these materials, including bioapatites, are often prone to damage during observation, including irradiation-induced crystallization. In the present study, high-resolution imaging at 200 kV acceleration voltage led to sample damage within a few seconds of observation ( Supplementary Fig. 5 ). At lower acceleration voltage, beam damage was slower but still noticeable ( Supplementary Fig. 6 ). Thus, confocal Raman proved a more suitable method to distinguish ordered versus disordered domains in the present work, especially for imaging microstructural features larger than ~1 μm. Nanoindentation and indentation fracture Reduced modulus ( E r ) and hardness ( H ) mapping on a yy cross-sectional plane of a spear sample ( Fig. 6a ) clearly indicate the presence of a steep mechanical gradient from the bulk, periodical region to the impact surface region, as previously found in dactyl smasher samples. E r values abruptly increase from 25–30 GPa in the bulk up to 65–70 GPa in the impact region, with peak values of 75 GPa measured immediately next to the outer surface. These gradients are directly correlated to variations in the phase chemistry: the softer bulk region is made of ACC (see associated Raman spectra in Fig. 5a ), the intermediate region corresponds to the transition from ACC to ACP (green colour on the indentation map), whereas the stiffest and hardest regions close to the impact surface are composed of FAP with small amounts of CAS (compare Fig. 6a with Fig. 5a ). The hardness mapping features’ identical trends, with H increasing from 1–1.5 GPa in the bulk up to 6–6.5 GPa in the impact region. To correlate further the mechanical properties with the local crystallochemistry, high-resolution nanoindentation line scans were conducted across regions comprising the localized disordered zones (displayed in Fig. 3e and Fig. 5h ) as well as their adjacent crystalline domains. These scans with corresponding SEM images ( Fig. 6c,d ) indicate that in the localized disordered zones (highlighted in yellow, line 2), Young’s modulus gradient is less pronounced ( E r increasing from 50 to 55 GPa) than along line 1, where only crystalline domains are probed and where the modulus rapidly increases to maximum values of 75 GPa. Along line 2, as soon as the indents were placed on the crystalline regions, a sudden increase in E r is noticed, leading to values near the outer surface that are identical to those measured along line 1. 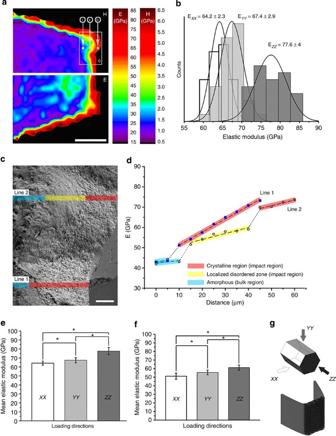Figure 6: Mechanical characterization of dactyl segments by nanoindentation. (a) (Scale bar, 100 μm) Reduced modulus (Er) and hardness (H) maps of a spear sample (yy cross-section). Latin numbers correspond to Raman spectra displayed inFig. 5a. (c,d) (Scale bar, 10 μm) High-resolution nanoindentation line scans. Line 1 (in the centre of the impact region) spans from the ACC bulk with a sharp transition to the FAP/CAS regions, whereas line 2 (along the extruded edge) encompasses the bulk (blue), the localized disordered zones (yellow) and the ordered FAP/CAS regions near the outer surface. (b)Erdistribution plots measured in the impact region normal to the three cross-sectional planes shown inFig. 1. (e,f) Average values ofErof a spear sample (e) (same data sets as in (b)) and of a smasher sample (f) in the impact region measured normal to thexx,yyandzzdirections, illustrating the mechanical anisotropy of the impact surface. *P<0.001. (g) Schematic representation of FAP crystallite orientation in the impact layer. Figure 6: Mechanical characterization of dactyl segments by nanoindentation. ( a ) (Scale bar, 100 μm) Reduced modulus ( E r ) and hardness ( H ) maps of a spear sample (yy cross-section). Latin numbers correspond to Raman spectra displayed in Fig. 5a . ( c , d ) (Scale bar, 10 μm) High-resolution nanoindentation line scans. Line 1 (in the centre of the impact region) spans from the ACC bulk with a sharp transition to the FAP/CAS regions, whereas line 2 (along the extruded edge) encompasses the bulk (blue), the localized disordered zones (yellow) and the ordered FAP/CAS regions near the outer surface. ( b ) E r distribution plots measured in the impact region normal to the three cross-sectional planes shown in Fig. 1 . ( e , f ) Average values of E r of a spear sample ( e ) (same data sets as in ( b )) and of a smasher sample ( f ) in the impact region measured normal to the xx , yy and zz directions, illustrating the mechanical anisotropy of the impact surface. * P <0.001. ( g ) Schematic representation of FAP crystallite orientation in the impact layer. Full size image Given the preferred orientation of mineralized fibres in the impact region detected in both types of samples, the mechanical response was probed by indentation across three mutually perpendicular planes, with all indents performed in the extruded edge discussed above. A distribution plot and average values of a spear sample ( Fig. 6b,e ) show that the modulus is clearly anisotropic, with average values of 77.6±4.0 GPa normal to the free surface (zz plane), 67.4±2.9 GPa normal to the yy plane and 64.2±2.3 GPa normal to the xx plane. The anisotropic response for a smasher sample was also probed ( Fig. 6f ). While the absolute values are lower than the spearer sample, a similar anisotropic response is obtained and found to be statistically significant. Normal to the impact surface ( zz plane), the modulus is 61.1±3.1 GPa, whereas normal to the yy and xx planes, the modulus are 55.5±2.8 and 51.1±3.6 GPa, respectively. In summary, stiffness anisotropy is detected in both types of stomatopod’s dactyl segments. Fracture toughness values were evaluated using a methodology we previously developed for sponge biosilica [22] . A sharp cube-corner tip was selected for these experiments because of its ability to induce cracking at external loads one to two orders of magnitude lower than the Berkovich geometry. In addition, a high-load transducer allowing to perform indents from a few mN up to the N range was employed. A few indents were placed at each load (representative indentation fracture curves are provided in Supplementary Fig. 7 ), which were subsequently observed by FESEM to determine the fraction of cracked corners. With this method, a nucleation load P c corresponding to the critical load for sharp indentation cracking is obtained (defined as the fraction of cracked corners of 0.5), from which a value of fracture toughness at initiation can be evaluated using a micromechanical model presented in Lawn [23] . In comparison to the H and E values combination, a clearer contrast between the species is observed, with a P c value for the smasher club of 145 versus 21.4 mN for the spearer appendage ( Fig. 7a ). This translates into fracture toughness values of 2.02 and 1.47 MPa·m 1/2 . To complement these fracture data, we also acquired Raman spectra in the impact regions. A Raman shift doublet near 3,000 cm −1 corresponding to chitin, as well as minor bands in the range 1,300–1,400 cm −1 also attributed to chitin [24] , were detected in the smasher dactyl club impact region but not in the spearer species ( Fig. 7b ). 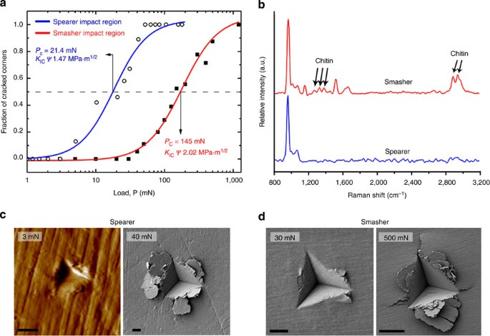Figure 7: Indentation fracture analysis of the dactyl appendage’s impact regions. (a) Cracking frequency at indent corners versus peak load (cube-corner tip). (b) Representative Raman spectra from 800 to 3,200 cm−1wavenumber acquired near the indents. Chitin is detected in the impact region of the smasher dactyl club, but not of the spearer dactyl appendage. (c) (Scale bar, 1 μm) Scanning probe microscope and SEM micrographs of residual indents on spear samples after indentation peak loads of 3 mN (left) and 40 mN (right). (d) (Left scale bar, 1 μm; right scale bar, 10 μm) SEM micrographs of residual indents on smasher samples after indentation peak loads of 30 mN (left) and 500 mN (right). Figure 7: Indentation fracture analysis of the dactyl appendage’s impact regions. ( a ) Cracking frequency at indent corners versus peak load (cube-corner tip). ( b ) Representative Raman spectra from 800 to 3,200 cm −1 wavenumber acquired near the indents. Chitin is detected in the impact region of the smasher dactyl club, but not of the spearer dactyl appendage. ( c ) (Scale bar, 1 μm) Scanning probe microscope and SEM micrographs of residual indents on spear samples after indentation peak loads of 3 mN (left) and 40 mN (right). ( d ) (Left scale bar, 1 μm; right scale bar, 10 μm) SEM micrographs of residual indents on smasher samples after indentation peak loads of 30 mN (left) and 500 mN (right). Full size image The predatory success of stomatopods is intimately linked to the mechanical efficiency of their dactyl spear and club-like dactyl modifications, and the impact surface is especially important in inflicting large forces during feeding and defence. The present data provide important refinements to the crystallochemistry of the phases present in the impact region of stomatopod dactyl segments. Raman spectroscopy provides clear evidences, in both types of appendages, of the amorphous-to-crystalline transition of the apatite phase, which from the peak location (965 cm −1 ) ( Fig. 5a,b ) appears to be FAP [14] as opposed to HAP. This Raman shift of the phosphate peak location towards FAP in the impact region is clearly visualized in the map displayed in Fig. 5g . Finally, the presence of FAP as the dominant crystalline phase is corroborated by high-resolution EDS mapping ( Fig. 4 ) as well as by EPMA quantitative elemental analysis ( Supplementary Table 1 ), which show fluorine enrichment in the impact region that correlates with higher phosphorous and calcium distributions. These variations in phase chemistry and ordering are directly correlated to mechanical gradients. As the main phase from the bulk to the impact surface transitions from ACC to ACP to FAP, the dactyl clubs become stiffer and harder. Localized disordered zones in the impact region, however, appear significantly softer and less stiff ( Fig. 6c,d ). Given that maximum principal stresses during impact are predicted to be located near the impact/periodic region interface [2] , this may imply a mechanical damping role for these localized, more compliant disordered zones. The usage of phosphate over carbonate, which is the common mineral-building block synthesized by many invertebrates for most of their protective structures, is unusual. In fact, the occurrence of apatite in general is uncommon among invertebrates [25] , [26] , although FAP was recently reported in the outer crown of crayfish mandibles [11] , which also displayed a carbonate-to-phosphate transition followed by an amorphous-to-crystalline conversion of the apatite phase. These observations suggest that the synthesis of apatite in the biotools or teeth of invertebrates, especially crustaceans, may be more widespread in nature than previously recognized. From a mechanical and physicochemical perspective, there are several advantages for the animal to process FAP for their mechanically active appendages. First, as a consequence of its more compact structure and higher mechanical stability, FAP appears to be slightly stiffer and stronger than HAP, as reported by Enax et al. [27] who measured higher values of E r and H in FAP single crystals in comparison to HAP. Other evidences of higher modulus in FAP have been obtained using nanomechanical [28] and acoustic emission microscopy techniques [29] . Furthermore, fluoride ions have been reported to enhance the matrix protein–mineral interaction and to facilitate packing and organization of apatite crystal arrays [30] . Ab initio computational studies of various apatites have also suggested that FAP has a slightly higher elastic and bulk modulus than HAP [31] . Perhaps more significant, fluorination is well established to decrease the solubility of apatite in water by several orders of magnitude [32] , [33] , resulting in its extensive incorporation in the jaws of aggressive marine predators such as sharks [34] , [35] . Likewise, the impact surface of stomatopod dactyl segments must be shielded from chemical dissolution to fulfil their function, and thus it is not surprising that FAP is chemically favored over HAP. Even more peculiar than FAP is the occurrence of a sulphated biomineral in the impact region in both types of dactyl segments. To the best of our knowledge, a sulphated mineral had not been previously reported in load-bearing biological materials. In comparison to phosphates and carbonates, sulphates are not commonly synthesized by living organisms, and when they are, they serve highly specific function such as in the statoliths of jelly fish (CaSO 4 ·2 H 2 O, gypsum) or in certain algae (BaSO 4 , barite) [36] . This rare occurrence of CAS begs the question of its role in stomatopod dactyl segments. Confocal Raman imaging provides key insights to answer this question. A higher sulphate concentration in the form of gypsum is concomitantly accompanied with a higher crystallinity of the fluoroapatite phase (compare Fig. 5e,h ). Thus, the data suggest that there is a direct correlation between sulphate content and FAP crystallinity, indicating that CAS may play a role in the disordered-to-ordered transition of FAP. To test this hypothesis, we performed ab initio computations of interfacial FAP/CAS relationships. Using the COMPASS force field package [37] , the three structures were first constructed and verified against established crystal structure lattices [38] . Various interfacial crystallographic relationships were tested, and the [100] FAP //[100] CAS gave the best interfacial lattice matching ( Fig. 8 ). Computations indicated that the interface can be stabilized by a network of interphase hydrogen bonding between FAP and gypsum, suggesting that hydrogen bonding plays an important role in providing binding strength at the interface. The computations, which are based on the density functional theory whose capabilities have been used extensively to predict H-bonding network [39] , [40] , also show that the hydrogen bond network is mediated through the gypsum water molecules, suggesting that the hydration state of sulphate plays a specific stabilization role at the interface. To compare the influence of fluoride ions on interface stability, we computed the bond length and bond energies of both FAP/CAS and HAP/CAS interfaces. For CAS/FAP, we found that the H–F hydrogen bond length interface is 1.95 versus 2.06 Å for the H–OH bond length of the CAS/HAP interface, and that the binding energy of the FAP/CAS interface is 2 kCal mol −1 stronger per hydrogen bond. Taken together, these data imply that CAS could play a templating role for the disordered-to-ordered transition of FAP, thus explaining the co-localization of crystalline FAP with CAS. One possible two-step mechanism for this phase transition would be for CAS to first stabilize ACP, which could then crystallize using the [100] CAS plane as a template that lowers the driving force for crystal nucleation and leads to a lower total free energy of the system. Epitaxial relationships between FAP and hydrated CAS have previously been observed for synthetically grown FAP crystals [41] . Moreover, the stronger binding energy of the FAP/CAS interface suggests that fluorine ions play a role to further optimize the stiffness and strength of the biomineralized complex near the outer impact surface. 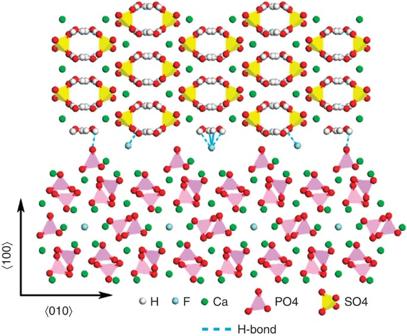Figure 8: FAP/CAS interfaces computed byab initiosimulations. Hydrogen bonding network is predicted to stabilize the interface along the [100] directions of both crystals. The binding energy in FAP/CAS is 2 kCal mol−1stronger per hydrogen bond than in hydroxyapatite (HAP)/CAS. Figure 8: FAP/CAS interfaces computed by ab initio simulations. Hydrogen bonding network is predicted to stabilize the interface along the [100] directions of both crystals. The binding energy in FAP/CAS is 2 kCal mol −1 stronger per hydrogen bond than in hydroxyapatite (HAP)/CAS. Full size image In addition to this chemical strategy, the mechanical response of dactyl segments’ impact regions is further tailored through preferred crystalline orientation, and this strategy is detected in both species. In the spearing type, polarized light and electron microscopy images indicate that FAP exhibits a polycrystalline texture, with the long crystallite axes oriented perpendicular to the impact surface. Further, evidence of the preferred orientation of FAP crystallites in the vicinity of the impact surface is supported by polarized Raman spectra acquired at 0° and 90° polarization angles relative to the free surface. The relative maxima of the ν 4 phosphate vibration mode (582 and 592 cm −1 ) match those measured on single HAP and FAP crystals ( Fig. 5c ) [19] , namely, the intensity ratio (I 582 /I 592 ) is less than unity at 90° and higher than unity at 0°, indicating that the c axes of FAP crystallites are oriented perpendicular to the impact surface. A final line of evidence confirming the preferred orientation of the FAP crystallites was obtained by inspecting the Raman spectral response from different directions, which showed variations in relative intensities between the major (965 cm −1 ) and the minor (1,075 cm −1 ) phosphate ν 1 bands when probed in the zz and yy orientations, respectively ( Supplementary Fig. 3 ). These variations in relative intensities were further corroborated by computing the Raman vibration modes using ab initio computations ( Supplementary Note 2 ). In the dactyl clubs from the smashing species, synchrotron X-ray diffraction data previously showed that the apatite crystals were preferentially oriented with their c -axis perpendicular to the impact surface [2] . FAP has a hexagonal crystal structure with an anisotropic stiffness tensor, resulting in a higher modulus in the direction normal to the basal plane (parallel to the lattice c -axis) than normal to the prismatic planes (parallel to the lattice a and b axes). Stiffness constants of FAP have been computed by ab initio [31] and force field [42] simulation methods. The absolute values of computed FAP stiffness constants, in the range 126–150 GPa for C 11 and 167–180 GPa for C 33 —which would correspond to the moduli if the measurements were ideally carried out normal to the basal and prismatic crystal planes, respectively—are clearly higher than the modulus values of stomatopod’s dactyl segments. This is likely related to the polycrystalline nature of the FAP crystals and to the presence of a thin organic matrix in the dactyls, which can lead to inter-crystalline sliding during indentation measurements. Meaningful comparisons between computations and experiments, however, can still be obtained by comparing the stiffness constant ratio C 33 / C 11 . Menéndez-Proupin et al. [31] reported a C 33 / C 11 ratio of 1.33, while Mkhonto and De Leeuw [42] obtained a ratio of 1.17. For the spearer sample, the ratio of the reduced modulus normal to the impact surface over the reduced modulus parallel to the impact surface E zz / E xx is equal to 1.21, whereas for the smasher sample the ratio is E zz / E xx =1.18 ( Fig. 6b,e,f ). The moduli ratios, close to 1.20 for both species, are within the range predicted by computer simulations on single crystals, confirming the textured orientation of FAP crystals in the impact region with the basal plane oriented parallel to the impact-free surface. Experimental measurements of the C 33 / C 11 ratio of FAP single crystals have also been carried out using an ultrasound technique [42] , and values in the range 1.22–1.25 were reported, again close to the present experimental data. It should be mentioned that the ratios E zz / E yy are significantly smaller (1.15 and 1.10 for the spearer and the smasher, respectively), which can be attributed to two main sources. First, the xx plane in our experiments is perpendicular to the yy plane, whereas in the hexagonal crystal structure the prismatic planes are oriented at 60° from each other. Even if the FAP crystals were perfectly oriented with the c -axis normal to the zz measurement plane, either the xx or the xx planes would not coincide to a main prismatic crystal plane. Second, it is likely that not all grains are perfectly oriented with the c -axis normal to the impact surface, resulting in less elastic asymmetry during measurements because indentation experiments are actually carried out at an angle from the principal crystal axes. While optimized hardness and modulus are important for maximizing impact forces during prey knocking, an additional biomechanical requirement is a fracture resistance in the impact region that is high enough to prevent permanent microdamage to the appendages. Since the microscopic size of the impact region (<100 μm) precludes the usage of standard fracture toughness specimens, as has, for instance, been done for other biominerals such as conch shells [43] or bone [44] (even ‘miniaturized’ samples with sizes in the mm range are orders of magnitude larger than the dactyl appendages’ impact regions), fracture toughness was assessed by indentation fracture [22] . The method is deemed suitable as a comparative assessment of the fracture resistance. (Comprehensive fracture toughness studies could perhaps be conducted by machining microscale beam specimens, and subsequently testing them by bending with a nanoindenter or AFM. However, nanoscale sample machining of biological samples with techniques such as focus ion beam currently does not allow to prepare damage-free specimens of suitable size.) The fracture data, summarized in Fig. 7 , indicate a better tolerance to damage for the smasher species with fracture toughness values of ~2 versus 1.5 MPa.m 1/2 for the spearer species. The data should be considered with a certain level of caution because the R curve behaviour, namely, the increase in fracture resistance with crack propagation due to the building up of a fracture process zone [45] , is not captured by indentation fracture. Hence, the present values should be regarded as fracture toughness values at initiation. Nevertheless, the contrast in the critical nucleation load P c between the two species is evident (145 mN for the smasher versus 21.4 mN for the spearer, see also post-indentation fracture images in Fig. 7c,d ) and strongly suggests a relation with evolution pressures and hunting strategies. Whereas the spearer species does in some instance use its dactyl segments to punch its preys, its main approach is to grab them with the dactyl barbs, meaning that the appendage is more often loaded in a bending regime. In contrast, the smasher exclusively uses hard blows, which imposes a higher tolerance to impact damage for its club. Chitin was detected in the impact region of the smasher dactyl segments by Raman spectroscopy, but not in the spearer dactyl segments ( Fig. 7b ). Given the well-known role of thin organic phases in biocomposites in enhancing the fracture toughness [4] , [45] , the data suggest that over evolution timeline the smasher species, which evolved from the spearer ones [46] , has incorporated residual chitin in the impact region to increase the damage tolerance of its dactyl club. The presence of a small amount of chitin also explains the slightly lower hardness and modulus of the smasher clubs ( Fig. 6e,f ). Stomatopods have evolved a dual chemical and microstructural strategy for the outermost region of their dactyl segments to inflict high impact damage to their prey. The impact region of these remarkably robust appendages is composed of calcium phosphate with a finely-tuned phase transformation and chemistry. FAP crystallites in the impact region are oriented in a textured manner near the contact points to optimize impact forces perpendicular to the surface. The spatial correlation between CAS and a higher degree of FAP crystallinity, together with coherent lattice matching between the two phases as predicted by atomistic computations, suggests that FAP crystallization is enabled by the presence of CAS, an unusual biomineral that had not previously been reported in load-bearing biological materials. Ab initio computations indicate the FAP/CAS interface is mediated by hydrogen bonding, which is stronger than the HAP/CAS interfacial energy. This dual presence of FAP and CAS in the impact region, coupled with the increase in mechanical properties associated with higher crystallinity, denotes a composite strategy for strengthening appendages that are subjected to high impact forces. Our data also reveal that the smasher species has optimized its tolerance against fracture damage in the impact region through incorporation of thin inter-crystallite chitin as a toughening phase. Finally, this study provides insights for the synthetic fabrication of impact and wear-resistant fluoroapatite-based materials. Sample preparation Live smashing (Odontodactylus) and spearing ( Lysiosquilla) stomatopods were acquired from commercial sources in Singapore. The second thoracic appendages from each species were removed and stored in a −20 °C freezer. The dactyl segments from each appendage were embedded in an acrylic cold mounting resin (ClaroCit, Struers), sectioned with a slow-speed diamond saw, and polished with P1200/4000 grade of SiC paper and then 1 and 0.25 μm diamond paste. After each step, diamond paste particles and polishing debris were removed from the samples in an ultrasonic bath for 5 min. For anisotropic indentation studies, embedded samples were cut across two perpendicular planes using a slow-speed diamond saw ( Fig. 1 ). To ensure that the exposed surfaces were from the impact region (namely, less than a couple of microns from the original free surface), three mutually perpendicular planes were directly polished with a fine diamond paste without any coarse pre-polishing. The planes were oriented such that the normal to the zz plane was perpendicular to the impact surface, whereas the normal to the xx and yy planes was parallel to the impact surface ( Fig. 1 ). EDS and Raman mapping (described below) were acquired on the second halves of the yy planes. Microstructural imaging and characterization Polished cross-sections were imaged using a ZEISS Axio Scope A1 optical microscope in bright field, dark field and polarized light modes. The polarizer and analyser were fixed in cross-orientation and the images were acquired at a sample rotation of 0°, 45° and 90°. For FESEM, the dactyl segments were immersed in liquid nitrogen and immediately fractured in the lateral direction, and the cross-sections were coated with 5 nm Pt. Samples were examined with a FESEM (JEOL, 7600F) at a low 1 kV accelerating voltage. To prevent surface charging, lower secondary electron image as well as gentle-beam modes were used. EDS measurements were conducted on polished and carbon-coated dactyl samples ( yy planes), with a Bruker X-Flash energy dispersive spectrometer. EDS compositional maps were acquired at a 20 kV accelerating voltage. AFM images were acquired in the AC mode in air on polished cross-sectional samples using an Asylum MFP3D-Bio. Nanoworld SSS-NCH cantilevers with nominal resonant frequencies between 250 and 390 kHz were used. Cantilevers were driven slightly below resonance at a frequency of ~286 kHz and samples were scanned at a rate of ~1 Hz in a closed loop. TEM analyses were conducted on a powder sample ground from the impact region of the clubs, which was dispersed in ethanol and then carefully placed onto copper TEM grids. High-resolution imaging was carried out on a JEOL 2100F TEM operating at 200 kV. Because of the extreme instability and beam-induced crystallization of the samples under the beam, additional observations were conducted on a Carl Zeiss Libra 120 Plus BioTEM operating at an acceleration voltage of 120 kV. Electron diffraction patterns of particles distinguished in the bright-field mode were immediately recorded to minimize sample damage and crystallization of native amorphous regions under the beam. EPMA analyses Quantitative wavelength dispersive spectroscopy analyses were performed using a JXA‐8530F field emission gun electron probe X‐ray microanalyser. Point analyses were acquired using a 10 μm diameter defocused beam at a probe current of 10 nA and an accelerating voltage of 15 kV. Results were quantified using external calibration standards and a ZAF matrix correction procedure. Error on repeat analysis of standards was <2% of measured values. Raman spectroscopy and imaging Raman spectrometry of embedded and polished cross-sections was acquired with a Horiba LabRAM HR ( λ =785 nm) equipped with a × 100 microscope objective lens. Line mapping studies were performed along a straight line from the outermost layer of the bulk to the impact surface. Each Raman spectrum was acquired for 90 s and smoothed using the Horiba Labspec and OriginPro 8 software. Raman imaging was performed using a confocal Raman microscope (alpha300, WITec, Ulm, Germany) equipped with a frequency-doubled Nd:YAG laser excitation ( λ =532 nm) and a piezoscanner. The laser beam was focused on the sample through a Nikon 60X objective with a numerical aperture (NA) of 0.8 and a spot size of ~0.61 λ /NA. For imaging, an integration time of 0.3 s was used for acquisition, and pixels were separated by 0.5 μm. The spectra were acquired using a CCD detector (DU401A-BV, Andor, UK) placed behind the spectrometer (UHTS 300; WITec). The Spectroscopy Plus software (WITec) was used for measurements and WITec Project Plus for spectrum processing. The images were generated by integrating the intensity of the signal for the wavenumber ranges of phosphate (920–990 cm −1 ), sulphate (990–1,025 cm −1 ) and carbonate (1,040–1,125 cm −1 ). Regions that were subsequently characterized by indentation fracture were also probed by Raman spectroscopy in the range 800–3,200 cm −1 , selected to detect the potential presence of organic components. For these measurements, the average and baseline subtraction functions of the software were used to extract the average spectra and detect the possible presence of chitin. Nanoindentation Indentation studies were performed on three mutually perpendicular cross-sections ( Fig. 1 ) using a Triboindenter TI-950 Nanomechanical tester (Hysitron, Minneapolis, MN, USA) equipped with a Berkovich diamond tip. A peak force of 2 mN was used for the mapping mode and 1 mN for the 3D anisotropy studies. Each indentation experiment consisted of a 5 s loading and 5 s unloading cycle. In the mapping mode, indentations were performed on the xx cross-sectional plane of the impact region with indentation spacing of 15 μm. For the 3D anisotropy study, a series of 30 indents with a 10 μm interval were carried out. Indents were placed on the three cross-sectional planes defined above ( xx , yy and zz ), with P ii corresponding to indents perpendicular to the ii plane. Identical sample preparations were used for indentation fracture experiments. These tests were performed using a high-load 10 N transducer and a cube-corner diamond tip. Peak indentation loads were varied from 1 to 1,200 mN (1 to 200 mN for spearers and 10 to 1,200 mN for smashers based on preliminary observations). A total number of 46 indents and 64 indents for the spearer and smasher, respectively, were placed on the outermost regions of the samples. Following indentation, the indents were observed by FESEM with a JEOL 7600F microscope to visualize chipped and cracked corners. For the lowest load indents (<5 mN), the scanning probe microscopy mode of the nanoindenter was used to image the indents using a low-load (10 mN) transducer and a cube-corner diamond tip. The force point was set at 2 μN in the imaging mode. High-resolution line scan indentations were conducted using a cube-corner tip with 5 μm indent spacing and a ‘5–2–5’ s load function (loading–holding–unloading), with a maximum load of 1,500 μN. The tip was calibrated on fused quartz and polycarbonate standard samples for shallow and deep contact depths, respectively. Ab initio computations CAS, HAP and FAP structures were constructed using the COMPASS force field method [37] , which yielded good agreement with tabulated crystal structure data. Several hydrogen types were introduced based on the polar strength of the atom that the hydrogen was attached to. Due to a strong polarization effect produced by hydrogen bonding, the ab initio charge-bond increment scheme was adopted to describe the hydrogen bonding with good accuracy. Various interfacial models between CAS and FAP (or HAP) were constructed and the (100) planes gave the best lattice matching, thus leading to a coherent epitaxial interface. Raman vibration modes for the FAP crystals were performed using the CASTEP software package [47] , with a norm-conserving pseudo-potential, a kinetic energy cutoff of 630 eV in, and 1 × 1 × 2K sampling. The phonon modes were obtained by diagonalizing the dynamical matrix, in which the mass-reduced Fourier transformed into the force constant matrix. The force constants were computed by evaluating the response wavefunction with the perturbation theory. The Raman tensor was computed by the finite-difference method, that is the mode displacement derivatives of the polarizability tensor. The relative intensity- and polarization-dependent computed data were used to identify the modes responsible for the experimental peaks. How to cite this article: Amini, S. et al. Textured fluorapatite bonded to calcium sulphate strengthen stomatopod raptorial appendages. Nat. Commun. 5:3187 doi: 10.1038/ncomms4187 (2014).